Alba shapes the archaeal genome using a delicate balance of bridging and stiffening the DNA Architectural proteins have an important role in shaping the genome and act as global regulators of gene expression. How these proteins jointly modulate genome plasticity is largely unknown. In archaea, one of the most abundant proteins, Alba, is considered to have a key role in organizing the genome. Here we characterize the multimodal architectural properties and interplay of the Alba1 and Alba2 proteins using single-molecule imaging and manipulation techniques. We demonstrate that the two paralogues can bridge and rigidify DNA and that the interplay between the two proteins influences the balance between these effects. Our data yield a structural model that explains the multimodal behaviour of Alba proteins and its impact on genome folding. The genome inside organisms from all domains of life is very long compared with the size of the cell or compartment to which it is confined. Hence, genomic DNA needs to be tightly compacted to fit. To facilitate compaction cells utilize generic physical mechanisms such as molecular crowding and supercoiling [1] . In addition, cells synthesize architectural proteins that shape the structure of the genome [2] . Despite a general lack of homology between architectural proteins in organisms from different domains of life, the way they shape the genome seems highly conserved [2] . In bacteria architectural proteins such as HU and H-NS, respectively, shape the genome by inducing bends into DNA [3] or promoting loop formation between distant sites along the DNA [4] . All these proteins act jointly to organize and compact the genomic DNA into a structure referred to as the nucleoid. In eukaryotes the genome is organized by wrapping the DNA around histones, yielding a nucleosomal fibre [5] , [6] . This structure folds into a chromatin fibre, which is further organized into loops mediated by proteins such as CTCF and cohesin [7] , [8] , [9] . Mitochondria also harbour their own genome. The mitochondrial genome is not organized by histones, but instead by a set of small architectural proteins, analogous to the bacterial chromatin [10] , [11] . Relatively little is known about the architectural properties of the proteins that shape the genome in archaea [12] , [13] . Archaea are unicellular organisms that share the DNA replication, transcription and translation machinery with eukaryotes [14] , and are therefore often used as a model for the more complicated eukaryotic systems. Analogous to bacteria, archaea lack a nucleus and their genome is organized into a nucleoid, using strategies of both eukaryotes and bacteria. Several archaeal branches exist of which the main two are the Euryarchaea and the Crenarchaea. Euryarchaea encode legitimate homologues of eukaryotic histone proteins [15] , while Crenarchaea generally lack histones and encode architectural proteins that use mechanisms as observed in bacteria [12] , [16] . Alba (Acetylation Lowers Binding Affinity) is one of the most abundant and highly conserved non-specific double-stranded DNA-binding proteins found throughout the archaeal domain [13] , [17] , [18] (~4% of the cellular protein in Sulfolobus shibatae [19] ), making it a key candidate to be involved in chromatin organization. Alba is a small protein (~10 kDa per subunit) that forms dimers in solution; larger multimeric forms of the protein have not been reported [20] , [21] . The crystal structure of the protein has been known for over a decade [22] , while an Alba–DNA co-crystal structure was resolved only recently [23] . Alba has been suggested to have two distinct structural effects on DNA depending on the protein:DNA stoichiometry. At low stoichiometry (about one dimer per 15 bp) Alba is able to bring two duplexes of DNA together, while under saturating conditions (effectively one dimer per 5 bp) it binds cooperatively along the DNA [17] , [22] , [24] . Both types of effects rely on dimer–dimer interactions. Dimer–dimer interactions promote the cooperative side-by-side binding along DNA and have a direct impact on the ability to form a filamentous structure [24] . On the other hand, dimer–dimer interactions also appear to be responsible for bringing two DNA duplexes together [23] . A striking observation is that cooperative side-by-side binding along the DNA is affected by a mutation of the F60 residue [24] , which is also involved in the bridging dimer–dimer interactions [23] . Sulfolobus solfataricus encodes two distinct Alba proteins denoted Alba1 and Alba2 (ref. 21 ) (36% sequence identity and 63% sequence similarity). Alba2 has a 10-fold lower transcription level compared with Alba1 (ref. 21 ) and is expressed at ~5% of the Alba1 level in stationary phase [21] . Furthermore, Alba2 lacks the F60 residue that is responsible for the cooperative side-by-side binding of Alba1. Alba1 and Alba2 form obligate heterodimers, which have DNA-binding properties different from Alba1 homodimers. On the basis of this notion it has been proposed that tuning the fraction of heterodimers is a mechanism to modulate Alba-mediated genome organization in vivo [21] , [26] . Nevertheless, a comprehensive molecular model of the different modes of Alba binding, and the modulatory interplay between Alba1 and Alba2 in relation to genome organization is still unavailable. The action of architectural proteins has been studied in vitro for many years using conventional biochemical assays, as well as with single-molecule techniques more recently [27] , [28] . These techniques allow the visualization and manipulation of single DNA molecules interacting with single proteins and reveal the kinetics and dynamics of these interactions. Here we use a set of complementary single-molecule techniques to study the action and interplay of Alba1 and Alba2 on DNA. We characterize the structural changes of DNA upon Alba binding and investigate the physical properties of Alba–DNA complexes. On the basis of our results we propose a model that explains the concentration-dependent behaviour of Alba1 and its modulation by Alba2. Visualizing Alba–DNA interactions To investigate the architectural properties of Alba proteins, Alba–DNA complexes were visualized using atomic force microscopy (AFM) at different protein:DNA stoichiometries. A series of representative images for each stoichiometry is shown in Fig. 1 . The complexes were classified by visual inspection of the AFM images into ‘open’, ‘bridged’ or ‘condensed’ (Methods section) and counted for different stoichiometries ( Supplementary Fig. S1 ). 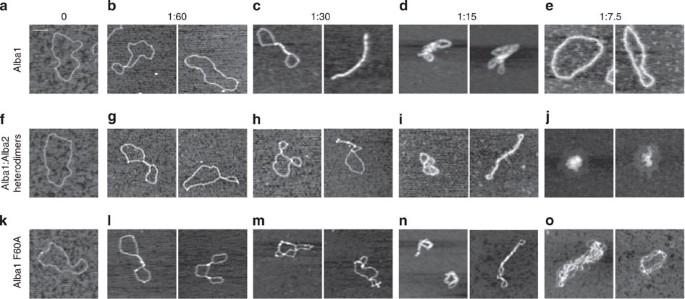Figure 1: Alba bridges and compacts DNA. Representative images of Alba–DNA complexes visualized by AFM. Nicked pRD24 plasmids are incubated at different stoichiometries (indicated as dimer:bp) with different Alba proteins. (a–e) Alba1 forms bridges at 1:60 and 1:30 ratios, condenses molecules at a 1:15 ratio and forms stiff open DNA molecules at 1:7.5 ratio. (f–j) Alba1:Alba2 heterodimers form bridged protein–DNA complexes at 1:60, 1:30 and 1:15. However, at 1:7.5 ratio DNA molecules are highly condensed, and do not show a stiffened configuration as Alba1. (k–o) Alba1 F60A dimers are able to form bridges between DNA duplexes at all different concentrations. Alba1 F60A and Alba2 both lack the crucial F60 residue and its equivalent. The sequence identity of the α1-helix responsible for dimer–dimer interactions in both proteins is only 36%, which might explain the differences between Alba1 F60A homodimers and Alba1:Alba2 heterodimers. Scale bar, 100 nm. Figure 1: Alba bridges and compacts DNA. Representative images of Alba–DNA complexes visualized by AFM. Nicked pRD24 plasmids are incubated at different stoichiometries (indicated as dimer:bp) with different Alba proteins. ( a – e ) Alba1 forms bridges at 1:60 and 1:30 ratios, condenses molecules at a 1:15 ratio and forms stiff open DNA molecules at 1:7.5 ratio. ( f – j ) Alba1:Alba2 heterodimers form bridged protein–DNA complexes at 1:60, 1:30 and 1:15. However, at 1:7.5 ratio DNA molecules are highly condensed, and do not show a stiffened configuration as Alba1. ( k – o ) Alba1 F60A dimers are able to form bridges between DNA duplexes at all different concentrations. Alba1 F60A and Alba2 both lack the crucial F60 residue and its equivalent. The sequence identity of the α1-helix responsible for dimer–dimer interactions in both proteins is only 36%, which might explain the differences between Alba1 F60A homodimers and Alba1:Alba2 heterodimers. Scale bar, 100 nm. Full size image At protein:DNA ratios of 1:60 and 1:30 dimer:bp Alba1 binding resulted in the formation of intramolecular bridges. At 1:30 dimer:bp most Alba1–DNA complexes are bridged (60%), of which most contained a single protein patch extending over part of the DNA molecule ( Fig. 1c , left), and even some of the DNA molecules were found to be completely bridged (14% of all molecules) ( Fig. 1c , right). Both features suggest DNA-induced cooperative bridging, which is enhanced by the formation of stable bridges. At increased protein–DNA ratios (1:15 dimer:bp) multiple sites of bridging are commonly seen within the same molecule, causing the DNA molecule to condense ( Fig. 1d ). At even higher protein:DNA ratios (1:7.5 dimer:bp) DNA molecules attained an open appearance ( Fig. 1e ), suggesting stiffening of the DNA by cooperative side-by-side binding along the DNA molecule as reported previously [24] . To investigate the role of the dimer–dimer interface in cooperative side-by-side binding we studied Alba1:Alba2 heterodimers. As the Alba2 subunit lacks the conserved F60 dimer–dimer interface, we would expect cooperativity to be suppressed. Binding of the heterodimers at protein–DNA ratios of 1:60 and 1:30 dimer:bp resulted in intramolecular bridges as seen with the wild-type Alba1 ( Fig. 1g ). However, the images show that the heterodimers do not exhibit the same cooperative behaviour as Alba1 homodimers, as none of the molecules were completely bridged. At increased protein:DNA ratios (1:15 dimer:bp) relatively more bridged and condensed molecules were observed ( Fig. 1i ). In stark contrast with Alba1 homodimers, at a concentration of 1:7.5 dimer:bp, all DNA complexes were strongly condensed instead of stiffened ( Fig. 1j ), pointing, as expected, to a reduction in cooperativity between adjacent dimers in comparison with the Alba1 homodimers. As the F60 residue has been shown to be responsible for cooperative side-by-side binding, we studied DNA-binding properties of the Alba1 F60A mutant [24] . Binding of the Alba1 F60A mutant at concentrations of 1:60 and 1:30 dimer:bp yielded intramolecular bridges comparable to the Alba1:Alba2 protein–DNA complexes ( Fig. 1 l ). DNA condensation was observed at increased protein:DNA ratios ( Fig. 1 n ). Stiff and open molecules as with the wild-type protein were never observed. These results confirm the importance of the dimer–dimer interactions for cooperative side-by-side binding and the essential role of residue F60 therein. The reported AFM experiments provide us with snapshots of Alba–DNA complexes at different stoichiometries. However, to obtain a quantitative understanding of the DNA binding and bridging properties of Alba, we performed dynamic measurements on single DNA molecules in solution using several different optical trapping configurations. Mechanical properties of Alba1–DNA complexes First we investigated the effect of Alba1 on the physical properties of single DNA molecules. In these experiments, a DNA molecule is captured between two optically trapped beads and gradually stretched while the force on the molecule is recorded ( Fig. 2a ), resulting in a force–distance (FD) curve. First a FD curve of bare DNA is measured as a reference ( Fig. 2b , black curve). Subsequently, the same molecule is incubated with Alba1, and a new FD curve is recorded to measure the effect of Alba1 on the physical properties of the DNA ( Fig. 2b , green and magenta curves). At low protein concentrations (1–100 nM) intersegmental bridging was observed (as reflected in numerous peaks in force at distances far below the contour length), which could be disrupted by applied force in some cases ( Fig. 2b , green curve). However, in most cases, bridges could resist forces even up to 400 pN (maximum force that can be applied in our instrument), pointing to extremely stable bridging interactions. At concentrations where the DNA molecules were saturated with Alba1 (>100 nM) no bridging was observed ( Fig. 2b , magenta curve). Instead, at low extension less force was required to stretch the protein–DNA ( Fig. 2b , magenta versus black curve), which indicates that less entropic energy is present and that the binding of Alba1 stiffens the DNA molecule. To quantify the observed stiffening, FD curves were recorded over a range of protein concentrations (1–2,000 nM) and fitted with the extensible worm-like chain model (eWLC) model (Equation 1). The contour length ( L C ) and the stretching modulus ( K 0 ) were found to be constant over the measured concentration range ( Supplementary Table S1 ). However, the persistence length ( L P ), which is a measure for the flexibility of the DNA, increased up to a five-fold higher value at protein concentrations >100 nM ( L P =260±30 nm for 2 μM Alba1 compared with L P =49±2 nm for bare DNA, see Fig. 2c , black circles). The increase in persistence length confirms that protein binding induces stiffening of the DNA as was observed in our AFM experiments ( Fig. 1e ). To investigate the impact of Alba on the twist parameters of DNA (twist–stretch coupling and torsional stiffness) the twistable WLC model (Equation 2) was fitted to the FD curves measured at 2 μM Alba1, obtaining g 0 =−560±100 pN nm, g 1 =19±6 nm and F C =31±7 pN ( N =10). These values show no deviation within the error from the values of bare DNA [29] , indicating that Alba1 does not change the twist–stretch coupling of DNA. 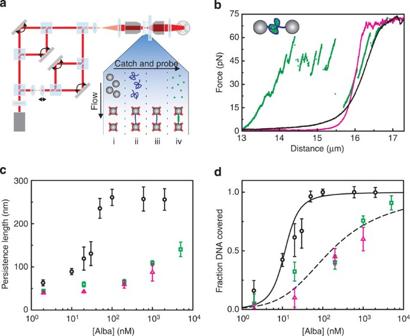Figure 2: Characterization of Alba–DNA binding by DNA micromanipulation experiments. (a) Schematic of the optical trapping setup used for both single and dual DNA experiments. Four optical traps are generated using a single laser. Each trap is steerable by a piezo-driven mirror. DNA molecules are caught (i–ii), tested (iii) and measured (iv) in a multi-channel flow cell. (b) FD curves of individual λ DNA molecules without protein (black curve), in the presence of 10 nM (green curve) and 2 μM Alba1 (magenta curve). At 10 nM Alba1, the FD curve shows several peaks in the force before the molecule is fully extended, indicating that the DNA molecule is bridged (cartoon inset). At a concentration of 2 μM Alba1 the DNA molecule is stiffened (magenta curve). (c) The persistence length (LP) measured at different protein concentrations of Alba1, Alba1 F60A and Alba1:Alba2 heterodimers (black circles, green squares and magenta triangles, respectively). The persistence length is obtained by fitting FD curves with the eWLC model (Equation 1). The value for naked DNA was found to beLp=49±2 nm. Error bars represent standard error of the mean. (d) The fractional coverage of Alba1, Alba1 F60A and Alba1:Alba2 heterodimers as a function of the concentration (black circles, green squares and magenta triangles, respectively). The Alba1 data points are fitted by the cooperative binding McGhee-von Hippel model (K=380±100 nM−1,ω=260±80, solid line). The model with similar parameters butω=1 (dashed line) describes the data points of Alba1 F60A and the Alba1:Alba2 heterodimers well, confirming the lack of cooperativity. Error bars represent the standard error of the mean. Figure 2: Characterization of Alba–DNA binding by DNA micromanipulation experiments. ( a ) Schematic of the optical trapping setup used for both single and dual DNA experiments. Four optical traps are generated using a single laser. Each trap is steerable by a piezo-driven mirror. DNA molecules are caught (i–ii), tested (iii) and measured (iv) in a multi-channel flow cell. ( b ) FD curves of individual λ DNA molecules without protein (black curve), in the presence of 10 nM (green curve) and 2 μM Alba1 (magenta curve). At 10 nM Alba1, the FD curve shows several peaks in the force before the molecule is fully extended, indicating that the DNA molecule is bridged (cartoon inset). At a concentration of 2 μM Alba1 the DNA molecule is stiffened (magenta curve). ( c ) The persistence length ( L P ) measured at different protein concentrations of Alba1, Alba1 F60A and Alba1:Alba2 heterodimers (black circles, green squares and magenta triangles, respectively). The persistence length is obtained by fitting FD curves with the eWLC model (Equation 1). The value for naked DNA was found to be L p =49±2 nm. Error bars represent standard error of the mean. ( d ) The fractional coverage of Alba1, Alba1 F60A and Alba1:Alba2 heterodimers as a function of the concentration (black circles, green squares and magenta triangles, respectively). The Alba1 data points are fitted by the cooperative binding McGhee-von Hippel model ( K =380±100 nM −1 , ω =260±80, solid line). The model with similar parameters but ω =1 (dashed line) describes the data points of Alba1 F60A and the Alba1:Alba2 heterodimers well, confirming the lack of cooperativity. Error bars represent the standard error of the mean. Full size image Cooperative binding of Alba1 The DNA-binding kinetics of Alba1 on DNA can be extracted from the amount of Alba1 bound to the molecule as a function of concentration. The persistence length of the Alba1-coated DNA molecules reached its maximum around 100 nM and stayed constant up to 2 μM, indicating that the DNA is saturated ( υ =1). The fractional DNA coverage is calculated from the persistence length as a function of the Alba1 concentration using Equation 5 ( Fig. 2d , black circles). Using the reported value of the binding site n =5 bp [22] , [23] , the McGhee-von Hippel model (Equation 6) fits well to the calculated coverage levels of Alba1–DNA binding ( Fig. 2d , black line). The fit yields an association constant K =(4±1)·10 2 nM −1 and a cooperativity factor ω =(3±1)·10 2 . The value of ω 1 confirms the cooperative binding of Alba1 along DNA, as observed in AFM experiments and shown in earlier work [24] . Alba1:Alba2 heterodimers lack cooperative binding behaviour To investigate the functional differences and interplay between the two homologous Alba proteins we characterized the effect of Alba1:Alba2 heterodimers on the mechanical properties of the DNA. The functional and structural consequences of Alba1:Alba2 heterodimer formation are best quantitatively addressed in the absence of Alba1 and Alba2 homodimers. When mixed at a 1:1 ratio—as in our experiments—only heterodimers are formed [21] . We find that these heterodimers increase the persistence length of DNA ( Fig. 2c , magenta triangles), yet, to a lower extent than Alba1. The impact of the Alba1:Alba2 heterodimer on DNA is similar to that of the Alba1 F60A mutant, indicating that the F60 residue has an essential role in the cooperative increase of the persistence length ( Fig. 2c , green squares). To quantify this effect we determined the fractional coverage as a function of the protein concentration for both Alba1:Alba2 heterodimers and the Alba F60A mutant using Equation 5 ( Fig. 2d , magenta triangles and green squares, respectively). To investigate whether both binding curves are consistent with a loss in cooperativity, we plotted the McGhee-von Hippel model (Equation 6) using the derived binding affinity for Alba1 ( K =4 × 10 2 nM −1 ), the same binding site ( n =5 bp) but without cooperativity ( ω =1). The McGhee-von Hippel binding isotherm using these parameters describes both the Alba1:Alba2 heterodimer and Alba F60A binding curve very well ( Fig. 2d , dotted line), reaffirming that the F60 residue is responsible for side-by-side cooperative dimer–dimer interactions. We also assessed the influence of Alba1:Alba2 heterodimers within a context of abundant Alba1 homodimers (at a ratio of 1:20), which can be encountered in an in vivo situation [21] . However, at this ratio the small amount of Alba2 had no detectable effect on the cooperative formation of the Alba1 filament. Dynamics and structure of Alba-induced DNA bridging Alba1 induced intersegmental bridges at relatively low protein concentrations (1–100 nM) ( Fig. 2b , green curve). However, at saturating Alba1 concentrations (>100 nM), bridging was not observed. Intersegmental interactions might be reduced due to stiffening of the DNA molecule, thereby decreasing the chance of two DNA segments within the same molecule to come close enough to form bridges. To test whether this is the cause of the absence of bridges at high Alba concentrations, we probed interactions between two individual DNA molecules using a quadruple optical trap configuration. We incubated the DNA molecules in 1 μM Alba1 to fully saturate them and next brought the two Alba1–DNA into close proximity to allow bridge formation. No bridging events were observed showing that DNA coated with Alba1 is not able to interact with other Alba1–DNA filaments. This indicates that the absence of bridge formation is not caused by DNA stiffening, but instead the interaction domains required for bridging are not accessible when proteins have side-by-side interaction with adjacent proteins. As Alba1 F60A is capable of forming bridged protein–DNA complexes over a large range of concentrations the mutant is an ideal candidate to study Alba-induced bridges. Bridging dynamics and structure were investigated using two DNA molecules brought in close proximity that were subsequently incubated with Alba1 F60A (100 nM). After incubation, a force is applied to one end of a DNA molecule, exerting a uniform shearing force along all protein-mediated bridges ( Fig. 3a , inset). Typically the force on the opposite DNA molecule rises, indicating the existence of protein-mediated bridges ( Fig. 3a , black curve). Furthermore, sharp drops in the force can be registered as the bridges rupture. However, on most occasions the DNA bridges were able to resist shear forces of at least 400 pN ( Supplementary Fig. S2 ). It is interesting to note that Alba1 bridges are very stable compared with the bacterial DNA bridging protein H-NS, which was only able to withstand ~25 pN in shearing mode with equal pulling rate [4] . 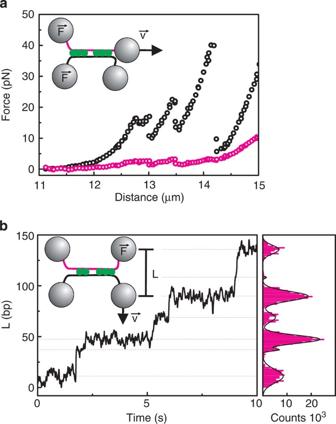Figure 3: Characterization of Alba-mediated bridges. Two DNA molecules are crossed and bridged by incubating in 100 nM Alba1 F60A. (a) Shearing experiment. One of the two DNA molecules is stretched with speedv(magenta strand), creating a uniform shearing force (F) over all the formed bridges. The force rises on the opposite molecule (black data points) and relaxes as protein–DNA complexes are ruptured. When the magenta DNA molecule is stretched to ~14.5 μm, the force also rises on the stretched molecule, possibly caused by bridges within the same molecule. (b) Unzipping experiment. A force up to 50 pN is built up over the first bridge between the two DNA molecules, by pulling perpendicular to the DNA molecules with speedv. As protein–DNA complexes are ruptured over time the length of DNA between the two beads (L) becomes larger in discrete steps. The histogram of the time trace is fitted with multiple Gaussians to find the step sizes (right panel), which represent the distance between two adjacent bridges. Figure 3: Characterization of Alba-mediated bridges. Two DNA molecules are crossed and bridged by incubating in 100 nM Alba1 F60A. ( a ) Shearing experiment. One of the two DNA molecules is stretched with speed v (magenta strand), creating a uniform shearing force ( F ) over all the formed bridges. The force rises on the opposite molecule (black data points) and relaxes as protein–DNA complexes are ruptured. When the magenta DNA molecule is stretched to ~14.5 μm, the force also rises on the stretched molecule, possibly caused by bridges within the same molecule. ( b ) Unzipping experiment. A force up to 50 pN is built up over the first bridge between the two DNA molecules, by pulling perpendicular to the DNA molecules with speed v . As protein–DNA complexes are ruptured over time the length of DNA between the two beads ( L ) becomes larger in discrete steps. The histogram of the time trace is fitted with multiple Gaussians to find the step sizes (right panel), which represent the distance between two adjacent bridges. Full size image To generate a force exclusively on the first protein-induced bridge, we performed unzipping experiments in which we pull perpendicular to the protein-induced DNA bridges ( Fig. 3b , inset). Forces up to 50 pN were required for bridge rupture. The rupture of a bridge causes the total DNA length between the two beads ( L ) to increase, leading to a decrease in the measured force. The experimental data show a clear stepwise increase of L , indicating rupture events of protein-mediated DNA bridges ( Fig. 3b , black curve). The amount of DNA that is released with the rupture of each protein-mediated bridge corresponds to the effective footprint of each bridge. As bridging the two DNA strands requires the faces of the helices to be aligned, the release in DNA is likely to correspond to an integer number of helical repeats (~10.5 bp). To extract the footprint of bridged patches with each rupture event, the histogram of the length ( L ) of each time trace is plotted and fitted with multiple Gaussians ( Fig. 3b , right panel). The distance between those peaks corresponds to the step size and is plotted in a histogram, which exhibits a distinct peak around ~20 bp, corresponding to a distance of two helical repeats ( Supplementary Fig. S3 ). This indicates that two adjacent bridges are less closely packed than found in the co-crystal structure, where the distance between two bridges is found to be a single helical repeat [23] . Our experiments have shown that Alba1 homodimers and Alba1:Alba2 heterodimers have distinct DNA-binding properties due to their difference in dimer–dimer interactions. McGhee-von Hippel analysis shows that Alba1 binds cooperatively along single DNA molecules, as suggested by previous data [17] , [24] , [30] . This cooperativity depends on the F60 residue, which is not conserved in the Alba2 paralogue. The fact that Alba1 F60A exhibits identical non-cooperative behaviour as the heterodimers ( Fig. 2d ) underlines the crucial role of the F60 residue in cooperative side-by-side binding. Besides having an important role in dimer–dimer stacking, the ability of Alba to bridge two DNA duplexes relies on a dimer–dimer interaction domain, which includes the F60 residue [23] . Apparently the dimer–dimer interface is responsible for two distinct structural effects on the DNA: bridging two DNA duplexes and stiffening by cooperative side-by-side binding. How can these two different binding modes be understood in one comprehensible model? A simple and straightforward generic model that would describe these data assumes that bridges can only be formed at low protein densities, when free DNA tracts are available for bridging. At higher protein densities no bridges can be formed. These types of effects are even more pronounced when protein binding is cooperative such that relatively low protein concentrations yield fully covered DNA (filaments). This model has been put forward to explain the DNA-binding properties of the H-NS-like proteins StpA and MvaT [31] , [32] . The H-NS-like proteins can bind side-by-side along a DNA molecule leading to DNA stiffening [31] , [32] . In the case of MvaT, it was shown that failure to form nucleoprotein filaments due to disturbed dimer–dimer interactions indeed enhances bridge formation [32] . In the case of these proteins no structural information of the proteins bound along DNA (stiffening) or between two DNA molecules (bridging) is available. H-NS and StpA differ from MvaT and the Alba proteins in their functional layout. H-NS and StpA have DNA-binding and multimerization domains separated. This is not the case for MvaT, where a point mutation can disrupt multimerization without affecting dimerization and DNA binding [32] . It is also not the case for Alba proteins where the same interface is involved in promoting side-by-side interactions along DNA and bridging interactions between DNA molecules [23] , [24] . Therefore, we propose a similar but more detailed model based on our experimental findings and the recent insights into the molecular basis of the dimer–dimer interactions. In this model Alba dimers can bind and alternate between two different orientations on the DNA, facilitating either bridging of two DNA duplexes or side-by-side binding of dimers ( Fig. 4a ). The cooperative side-by-side binding of Alba stiffens the DNA and consequently prevents bridges to form, due to the orientation of the dimer–dimer interaction domain in the direction of adjacent dimers along the DNA. This also explains the fact that two DNA molecules saturated with Alba1 proteins do not show any interaction when brought in close proximity. As Alba1:Alba2 dimers lack the conserved F60 residue at one side of the dimer, the dimer–dimer interactions along a single DNA duplex are limited to an interaction between two dimers ( Fig. 4b ) and consequently a long patch of closely packed dimers cannot be formed. Heterodimers are likely to be able to form bridges in three different configurations, depending on the orientation of the monomeric units within the bridged complex ( Fig. 4b ). The Alba1 F60A mutant confirms the important role of the dimer–dimer interactions on the DNA-binding properties of Alba, as it shows behaviour similar to that of the Alba1:Alba2 heterodimers ( Fig. 4c ). 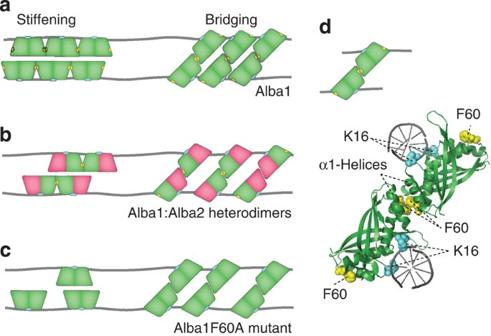Figure 4: Model of Alba-mediated stiffening and bridging. (a) Alba1 dimers can bind to the DNA in two different modes depending on their orientation on the DNA (cyan depicts DNA interaction domains). Dimers can either bind side-by-side along the DNA, stiffening the DNA, or interact with dimers on an adjacent duplex, yielding a bridged structure. The F60 residue (yellow) stabilizes dimer–dimer interactions and is responsible for cooperative side-by-side binding. (b) Alba1:Alba2 heterodimers can bind along the DNA but cooperative side-by-side binding is limited to a maximum of two dimers as only the Alba1 subunit contains the F60 residue. Bridged structures can be formed in three different configurations, depending on the orientation of the dimer in the bridged complex. (c) The Alba1 F60A mutant does not exhibit cooperative side-by-side binding along the DNA. Bridges can be formed, but are less stable compared with the Alba1 bridges. (d) Model of Alba1–DNA bridging interaction based on the Alba1 crystal structure (PDB accession code1H0X22) structurally aligned with the co-crystal structure of (Ape10b2)-dsDNA (PDB accession code2H9U23) using PyMol. Alba dimers interact with the minor groove of DNA (DNA-interacting K16 residues are shown in cyan). By hydrophobic interactions of the two α-helices and interactions of the F60 residues (yellow) two DNA duplexes are bridged. Figure 4: Model of Alba-mediated stiffening and bridging. ( a ) Alba1 dimers can bind to the DNA in two different modes depending on their orientation on the DNA (cyan depicts DNA interaction domains). Dimers can either bind side-by-side along the DNA, stiffening the DNA, or interact with dimers on an adjacent duplex, yielding a bridged structure. The F60 residue (yellow) stabilizes dimer–dimer interactions and is responsible for cooperative side-by-side binding. ( b ) Alba1:Alba2 heterodimers can bind along the DNA but cooperative side-by-side binding is limited to a maximum of two dimers as only the Alba1 subunit contains the F60 residue. Bridged structures can be formed in three different configurations, depending on the orientation of the dimer in the bridged complex. ( c ) The Alba1 F60A mutant does not exhibit cooperative side-by-side binding along the DNA. Bridges can be formed, but are less stable compared with the Alba1 bridges. ( d ) Model of Alba1–DNA bridging interaction based on the Alba1 crystal structure (PDB accession code 1H0X [22] ) structurally aligned with the co-crystal structure of (Ape10b2)-dsDNA (PDB accession code 2H9U [23] ) using PyMol. Alba dimers interact with the minor groove of DNA (DNA-interacting K16 residues are shown in cyan). By hydrophobic interactions of the two α-helices and interactions of the F60 residues (yellow) two DNA duplexes are bridged. Full size image Alba1 dimers, Alba1 F60A dimers and Alba1:Alba2 heterodimers are all able to form bridges at low protein:DNA ratios, which indicates that the F60 residue in the conserved dimer–dimer interface of Alba1 is not crucial for the formation of bridge structures. Indeed, the co-crystal structure of an Alba1 homologue from Aeropyrum pernix K1 (ref. 23 ) shows that the dimer–dimer interactions rely on hydrophobic interactions between the two α1-helices, which are additionally stabilized by the stacking interaction between the F60 residues ( Fig. 4d ). The Alba1 F60A mutant and the Alba1:Alba2 heterodimer are also able to form bridges, as the ability to bridge is warranted by the interactions of the two α1-helices ( Supplementary Fig. S4 ). Small differences in behaviour of the two types of dimers may be attributed to sequence differences between the α1-helices (only 36% sequence identity), leading to local variations in hydrophobicity along the helix that likely affect the strength of bridging. At relatively high protein concentrations, cooperative side-by-side binding of Alba1 yields stiff protein–DNA complexes. AFM images show that this results in stiff and open DNA molecules without any intersegmental bridges ( Fig. 1e ). At similar protein:DNA ratios, Alba1 F60A and Alba1:Alba2 heterodimers form condensed protein–DNA complexes by multiple bridged patches. In addition, McGhee-von Hippel analysis on the optical tweezers data demonstrated conclusively that the different behaviour of the Alba1:Alba2 heterodimers and the Alba1 F60A mutant is caused by a lack of cooperativity. These observations suggest that the Alba1 F60A mutant and the Alba1:Alba2 heterodimers cannot be packed closely along the DNA to form fully coated stiff filaments, due to the absence of the F60 residue in both units of Alba1 F60A dimers and in the Alba2 subunit of Alba1:Alba2 heterodimers. The ability of Alba to bridge two DNA duplexes suggests an important role in shaping archaeal chromatin structure. Architectural proteins that bridge DNA allow the formation of loops, which can functionally organize the genome [33] . In Escherichia coli , the genome is organized into topologically isolated domains [34] , [35] and the formation of these domains has been attributed to bridging/looping by H-NS [36] . Whether the archaeal genome is also organized in loops is to date unknown. If such a higher-order structure indeed exists, it could be facilitated by Alba-induced bridging. The dual binding mode of Alba can have an important role in shaping chromatin structure in vivo by tuning the balance between stiffened and bridged DNA. Such a dual binding mode has been reported for the bacterial chromatin protein H-NS (attributed to cis or trans binding of dimers [37] ) and been suggested to be important for gene regulation [38] , [39] . Although the molecular details of the binding mode of H-NS are different compared with Alba (the cis or trans binding is based on the binding mode of dimers instead of tetramers), the functional mechanisms could be very similar. However, whether Alba acts as a global gene regulator in a manner similar to H-NS [40] remains to be investigated. As Alba2 is expressed only at a few percents of Alba1, the majority of Alba in vivo will be in the form of Alba1 homodimers. Depending on the expression level of Alba1 and the resulting (local) Alba1 concentrations, dimers are able to form either stiffened regions of DNA or bridged duplexes. In addition, differential expression of Alba1 and Alba2 can tune the relative amount of Alba1:Alba2 heterodimers and interfere with the cooperative side-by-side binding of Alba1, making the stiffened regions of DNA more accessible. The interplay between Alba homodimers and heterodimers may thus have an important regulatory function in modulating gene accessibility, in addition to its role in genome organization. DNA and proteins The pRD24 plasmid (a pUC19 derivative, containing a Bpu10I recognition site inserted into the multiple cloning site) used for the AFM experiments was propagated in E. coli strain XL10 and purified (Qiagen plasmid midi kit). pRD24 was nicked by digestion with Bpu10l (Fermentas). The DNA used in the optical trapping experiments was made by labelling the 12-nucleotide long 5′ overhang of bacteriophage λ DNA (Roche) with dTTP, dGTP, biotin-14-dATP and biotin-14-dCTP using Klenow DNA polymerase exo− (Fermentas). The DNA was captured in the optical tweezers instrument between two streptavidin-coated beads (1.87 μm in diameter, Kisker) in buffer containing 10 mM Tris–HCl (pH 7.5), 200 mM NaCl, 1 mM EDTA and 3.5 mM DTT. Purification of the Alba1, Alba1 F60A and Alba2 proteins was carried out as described [21] , [22] , [24] . To obtain Alba1:Alba2 heterodimers the two proteins were mixed in a 1:1 ratio [21] . As Alba2 forms obligate heterodimers with Alba1 (ref. 21 ), this mixture will consist of Alba1:Alba2 heterodimers exclusively. Atomic force microscopy Alba–DNA complexes were formed by incubating 90 ng of nicked pRD24 with varying amounts of Alba proteins in 10 μl AFM buffer containing 40 mM Hepes (pH 7.5) and 25 mM NaCl for 30 min at room temperature (~23 °C). After incubation, this mixture was diluted 10-fold in 1 mM MgCl 2 and directly deposited onto freshly cleaved mica. After 40 s, the mica disc was rinsed with high-performance liquid chromatography water and dried with nitrogen gas. The AFM images were collected on a NanoScopeIII AFM (Digital Instruments, Santa Barbara, CA) using micro cantilevers (Olympus MCL-AC240TS-W2, resonance frequency 70 kHz, spring constant 2 N m −1 ). Images were obtained using tapping mode in air at 2 Hz and flattened using Nanoscope software (Veeco Instruments). The protein–DNA complexes were classified by visual inspection of the AFM images. Molecules with single DNA crossings or no crossings ( Fig. 1a ) were classified as ‘open’. Molecules with bridged patches, of which the length is longer than a single crossover of two DNA duplexes, were classified as ‘bridged’ ( Fig. 1g ). Molecules containing patches of more than two duplexes bridged ( Fig. 1d ) or highly compacted regions ( Fig. 1j ) were classified as ‘condensed’. Optical tweezers To perform DNA micromanipulation experiments, an instrument was designed and built, capable of manipulating four optical traps in three dimensions ( Fig. 2a ). Instead of time sharing three traps using an AOM [41] , we chose to use continuous traps (20 W, λ =1,070 nm YLR-20-LP IPG lasers GmbH) and rely on accurate piezo scanning mirrors rather than on motorized lenses [42] . The four optical traps enable manipulation and measurements on both a single DNA molecule (dual optical tweezers) and two DNA molecules (quadruple optical tweezers). The forces on the DNA molecules were measured by tracking bead displacement, using back focal plane interferometry on the trapping laser and using a second detection laser (140 mW, λ =980 nm; Power Technology Inc.) when using the quadruple optical trap. The measurements were carried out using a multi-channel laminar flow cell that permits rapid capture, testing and measurement of individual DNA molecules ( Fig. 2a ). After two individual DNA molecules have been caught, they were moved to a channel containing Alba in 10 mM Tris–HCl (pH 7.9), 1 mM EDTA, 3.5 mM DTT, 60 mM KCl, 10 mM MgCl 2 . In control experiments (bandshift assays) DNA-binding behaviour of Alba proteins did not differ in the absence or presence of 10 mM MgCl 2 (data not shown). The DNA molecules were incubated with Alba without applying tension for ~2 min. FD curves were recorded in ~30 s in the absence of flow. The resulting FD curves were highly reproducible under these conditions. The procedure of DNA catching and wrapping, switching buffers, incubation and force–distance measurement are all automated using a custom-written Labview software suite (National Instruments). All experiments were performed at room temperature (~23 °C). To quantify the properties of the measured DNA molecules and protein–DNA complexes, the FD curves are fitted to the eWLC [43] : This model gives a quantitative description of the mechanical properties of DNA in terms of the end-to-end distance ( d ) and its response to an applied force ( F ), which is dependent on the total length (contour length L C ), the flexibility (persistence length L P ) and the spring constant (stretching modulus K 0 ) of the DNA. To test whether the proteins have an effect on the twist–force response of the DNA, FD curves were also fitted to the twistable WLC, which describes how much the DNA unwinds as a function of the tension [29] : where C represents the twist rigidity and g ( F ) the force dependent twist–stretch coupling defined by parameters g 0 , g 1 and F C : To measure FD curves in experiments where bridging occurs, we fully extended the DNA molecule to remove these bridges and recorded the FD curve by decreasing the extension of the DNA molecule. If bridges within a molecule were too stable to be removed this molecule was discarded. Quantifying DNA coverage and binding kinetics At relatively low protein concentrations a fraction ( υ ) of DNA is covered by protein and the complementary fraction (1− υ ) consists of naked DNA. Assuming that each protein has an equal contribution to the increase of the DNA stiffness, the measured FD curve will be a linear combination of a FD curve of a saturated DNA molecule ( d saturated ( F )) and a FD curve of a bare DNA molecule ( d bare ( F )). An expression for the fractional coverage as a function of the persistence length is obtained by inserting the eWLC model (Equation 1, given that all parameters ( L C , K 0 and T ) are constant for all measured concentrations except for the persistence length ( L P ). This expression can be obtained for any other parameter as long as all other parameters are unaffected by protein binding [11] . The fractional coverage ( υ ) as a function of protein concentration ( c ) is fitted to the McGhee and von Hippel theory [44] , to obtain the kinetics on the protein–DNA interactions. In this theory, protein binding to DNA is described by the association constant ( K ), a cooperativity parameter ( ω ): the attractive or repulsive interactions between proteins binding to the DNA, and the effective binding site per protein in base pairs ( n ): where How to cite this article: Laurens, N. et al. Alba shapes the archaeal genome using a delicate balance of bridging and stiffening the DNA. Nat. Commun. 3:1328 doi: 10.1038/ncomms2330 (2012).